Binding of PHF1 Tudor to H3K36me3 enhances nucleosome accessibility The Tudor domain of human PHF1 recognizes trimethylated lysine 36 of histone H3 (H3K36me3). This interaction modulates the methyltransferase activity of the PRC2 complex and has a role in retention of PHF1 at DNA damage sites. We have previously determined the structural basis for the association of Tudor with a methylated histone peptide. Here we detail the molecular mechanism of binding of the Tudor domain to the H3K C 36me3-nucleosome core particle (H3K C 36me3-NCP). Using a combination of TROSY NMR and FRET, we show that Tudor concomitantly interacts with H3K36me3 and DNA. Binding of the PHF1 Tudor domain to the H3K C 36me3-NCP stabilizes the nucleosome in a conformation in which the nucleosomal DNA is more accessible to DNA-binding regulatory proteins. Our data provide a mechanistic explanation for the consequence of reading of the active mark H3K36me3 by the PHF1 Tudor domain. Human plant homeodomain (PHD) finger protein 1 (PHF1) is found in major nuclear regulatory complexes. PHF1 is an accessory component of the Polycomb Repressive Complex 2 (PRC2) that methylates lysine 27 of histone H3 and is required for gene silencing (reviewed in ref. 1 ). Upon genotoxic stress, PHF1 localizes to the sites of DNA damage through the association with DNA damage repair enzymes Ku70/Ku80 (ref. 2 ). PHF1 contains an N-terminal Tudor domain that binds to trimethylated lysine 36 of histone H3 (H3K36me3) [3] , [4] , [5] . This interaction inhibits the methyltransferase activity of PRC2 and has a role in the retention of PHF1 at the sites of double-stranded DNA (DS-DNA) breaks [3] . We have previously determined the structural basis of Tudor association with a peptide corresponding to the H3K36me3 tail (residues 31–40 of H3) [3] . However, the question remains as to how the Tudor domain binds to H3K36me3 in the context of the full nucleosome and even further, the chromatin fibre. This is an especially pressing question given that the position of this histone mark would place Tudor just adjacent to the nucleosome core, which may greatly alter the interaction. Although recent pioneering studies have begun shedding light on the mechanistic aspects for the association of effector domains with their target histone post-translational modifications (PTMs) on the nucleosome [6] , [7] , [8] , [9] , [10] , there is still a dearth of such reports. This is in large part due to experimental limitations. Most of the detailed structural information regarding the nucleosome complexes has been obtained by X-ray crystallography. However, because the N-terminal histone tails protrude from the nucleosome core and are solvent accessible and flexible, it has proven difficult to study interactions of effectors with the modified tails using crystallographic methods. Currently only four nucleosome/effector complexes have been successfully crystallized, and all reveal interactions with the particle core (and unmodified H4 tail in the case of the Sir3 BAH domain) [11] , [12] , [13] , [14] , [15] , [16] , [17] . As a result, various interactions with PTMs have been studied primarily using histone peptides, leaving a large gap in our knowledge of how these proteins bind to histone PTMs within the framework of the full nucleosome core particle (NCP). Nuclear magnetic resonance (NMR) spectroscopy is an ideal tool to address this question as it provides solution-state atomic resolution information and is very powerful in the detection and characterization of intermolecular interactions, even in very flexible constructs [18] , [19] . However, it remains challenging to produce modified nucleosomes in amounts sufficient for NMR analysis. Moreover, owing to the large size of the nucleosome/effector complexes, sophisticated labelling and advanced experimental methods are necessary to obtain quality data. Yet, progress is being made in this regard and exciting studies have recently demonstrated the influence of histone PTMs on the nucleosome and on the association with co-factors [7] , [9] . The issues with the NCP size and amount can be overcome by studying the nucleosome/effector interactions using Förster Resonance Energy Transfer (FRET), which requires only nanomolar concentrations of the NCPs. FRET has previously been used to demonstrate that the entry/exit regions of nucleosomal DNA transiently unwrap from and rapidly rewrap onto the histone core surface [20] , [21] , [22] . This phenomenon, which is often referred to as the DNA end ‘breathing’ motion, has a fundamental role in nucleosome remodelling, DNA replication and gene transcription. Here we describe the mechanism for binding of PHF1 Tudor to the H3K C 36me3-NCP and characterize the effect of this interaction on targeting a specific DNA site within the NCP by a protein effector. We show that in addition to recognizing H3K36me3, the Tudor domain associates with DNA, and such multiple contacts may account for a higher affinity of Tudor for the H3K C 36me3-NCP. Interaction of the PHF1 Tudor domain with the H3K C 36me3-NCP facilitates in vitro binding of the DNA-specific protein LexA to the DNA site that is inaccessible in the fully wrapped nucleosome, thus suggesting a shift in equilibrium towards a more open form of the nucleosome. Together, our findings provide a possible mechanistic explanation for the consequence of recognition of the H3K36me3 mark by the PHF1 Tudor domain. Tudor binds to the H3K C 36me3 nucleosome To determine the mechanism for recognition of the nucleosome by the Tudor domain of PHF1, we reconstituted the NCP carrying a methyl-lysine analogue (MLA) at position 36 of histone H3 (H3K C 36me3) ( Supplementary Fig. S1 ). We generated the H3(C110A)K36C mutant and subjected it to alkylation by (2-bromoethyl) trimethylammonium bromide to yield the N -methylated aminoethylcysteine derivative. The MLA histone was refolded with unmodified recombinant H2A, H2B and H4, and the resulting histone octamer was assembled onto a Widom 601 DNA sequence through slow desalting. Because the size of the H3K C 36me3-NCP/Tudor complex (~205 kDa) is beyond the limit of conventional NMR, we generated the double 2 D- and 15 N-labelled Tudor domain and characterized its binding to H3K C 36me3-NCP using 1 H, 15 N-transverse relaxation-optimized spectroscopy (TROSY)-heteronuclear single-quantum coherence (HSQC) experiments carried out at the elevated temperature of 310 K, on a 900 MHz spectrometer equipped with a cryogenic probe. The 1 H, 15 N-TROSY-HSQC spectra were collected on the free protein and in the presence of increasing concentrations of H3K C 36me3-NCP and overlayed ( Fig. 1a ). Titration of the H3K C 36me3-NCP up to 0.1 mM induced significant changes in the Tudor amide resonances, which could be grouped into the three sets. One set of resonances showed a substantial decrease in intensity and disappeared completely upon addition of 0.05 mM of the nucleosome. The second set of cross-peaks gradually moved, revealing the fast-to-intermediate exchange regime on the NMR timescale. The third set was perturbed to a lesser degree. At a 1:1 molar ratio there was, on average, an ~80% decrease in resonance intensity, indicating a robust interaction between Tudor and the H3K C 36me3-NCP. 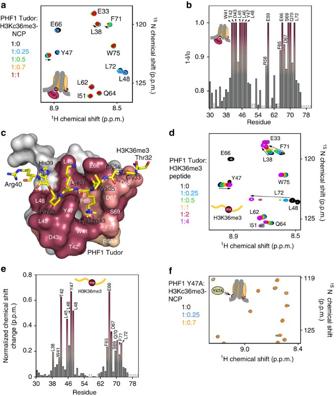Figure 1: Tudor interacts with the H3KC36me3-nucleosome. (a)1H,15N TROSY-HSQC spectral overlays of wild-type Tudor in the presence of increasing concentrations of H3KC36me3-NCP (molar ratio is shown to the left). (b) A plot of the decrease in resonance intensity (1−I/I0) induced by the H3KC36me3-NCP as a function of Tudor residue. Decreases of greater than 85, 90 and 96% are shown in tan, salmon and mauve, respectively. An asterisk indicates a missing or unassigned peak. The double asterisk indicates value below shown threshold. (c) Residues demonstrating significant decreases in resonance intensity are mapped onto a surface representation of Tudor with the H3K36me3 peptide shown as sticks in yellow. Residues of the H3K36me3 peptide and the Tudor domain are labelled using a three-letter code and a one-letter code, respectively. (d)1H,15N HSQC spectral overlays of wild-type Tudor in the presence of increasing concentrations of H3K36me3 peptide. (e) A plot of the extent of normalized chemical shift change induced by the H3K36me3 peptide as a function of Tudor residue, with changes greater than the average, average plus1/2or average plus 1 standard deviation shown in tan, salmon and mauve, respectively. An asterisk indicates a missing or unassigned peak. (f)1H,15N TROSY-HSQC spectral overlay of Y47A Tudor mutant in the presence of increasing concentrations of the H3KC36me3-NCP (molar ratio shown to the left). Figure 1: Tudor interacts with the H3K C 36me3-nucleosome. ( a ) 1 H, 15 N TROSY-HSQC spectral overlays of wild-type Tudor in the presence of increasing concentrations of H3K C 36me3-NCP (molar ratio is shown to the left). ( b ) A plot of the decrease in resonance intensity (1− I / I 0 ) induced by the H3K C 36me3-NCP as a function of Tudor residue. Decreases of greater than 85, 90 and 96% are shown in tan, salmon and mauve, respectively. An asterisk indicates a missing or unassigned peak. The double asterisk indicates value below shown threshold. ( c ) Residues demonstrating significant decreases in resonance intensity are mapped onto a surface representation of Tudor with the H3K36me3 peptide shown as sticks in yellow. Residues of the H3K36me3 peptide and the Tudor domain are labelled using a three-letter code and a one-letter code, respectively. ( d ) 1 H, 15 N HSQC spectral overlays of wild-type Tudor in the presence of increasing concentrations of H3K36me3 peptide. ( e ) A plot of the extent of normalized chemical shift change induced by the H3K36me3 peptide as a function of Tudor residue, with changes greater than the average, average plus 1 / 2 or average plus 1 standard deviation shown in tan, salmon and mauve, respectively. An asterisk indicates a missing or unassigned peak. ( f ) 1 H, 15 N TROSY-HSQC spectral overlay of Y47A Tudor mutant in the presence of increasing concentrations of the H3K C 36me3-NCP (molar ratio shown to the left). Full size image Plotting the intensity decrease (1− I / I 0 ) for each Tudor residue allowed us to identify the binding interface ( Fig. 1b ). Mapping the residues with rapidly disappearing amide signals onto the structure of the Tudor domain revealed an extensive patch at one of the open ends of the five-stranded β-barrel ( Fig. 1c , magenta). Many of these residues are directly involved in the interaction with H3K36me3 (ref. 3 ). Particularly, the aromatic cage, where trimethylated Lys36 is bound (PHF1 residues W41, Y47, F65 and F71), the adjacent hydrophobic patch underneath Pro38 of the peptide (PHF1 residues L45 and L46) and the acidic groove (PHF1 residues E66, D67 and D68) were significantly perturbed upon addition of the H3K C 36me3-NCP. This binding interface matched well to the binding surface mapped based on chemical shift changes observed in the 15 N-labelled Tudor domain as the H3K36me3 peptide was titrated in under similar conditions, that is, 310 K at 900 MHz ( Fig. 1d,e ). These results suggest that PHF1 Tudor binds to the methylated H3 tail of H3K C 36me3-NCP in a manner largely similar to how it associates with the histone peptide. However, several residues of PHF1 were perturbed by the nucleosome to a greater extent, specifically those that descend from the hydrophobic patch along the β2 strand of the barrel, as well as from the acidic patch along the β4 strand. In addition, R58 and E59 at the opposite end of the β-barrel were affected only upon binding to the H3K C 36me3-nucleosome, thus suggesting additional contacts with the intact NCP. Recognition of the trimethylated Lys36 residue remains the major driving force for binding of the PHF1 Tudor domain to H3K C 36me3-NCP. We tested the Y47A mutant of Tudor previously found to have impaired histone binding activity ( Fig. 1f ). Addition of H3K C 36me3-NCP to the 15 N-labelled Y47A mutant led to only a small and uniform decrease in resonance intensity, which is indicative of a very weak and non-specific association. These data reveal that a robust interaction with the NCP occurs only when Tudor is capable of binding to the H3K36me3 mark. Tudor has a high affinity for H3K C 36me3-NCP To assess the strength of the PHF1–NCP interaction, we carried out pulldown assays with GST-fusion Tudor domain ( Fig. 2 ). GST-Tudor was incubated first with increasing concentrations of H3K C 36me3-NCP and then with glutathione-agarose beads. After centrifugation, the nucleosome fraction bound to the protein was detected by western blot using an anti-H3 antibody ( Fig. 2a ). Densitometry analysis of the bound H3K C 36me3-NCP yielded an apparent K d of ~1.3 μM ( Fig. 2b ), and revealed that binding of the PHF1 GST-fusion Tudor domain to H3K C 36me3-NCP is stronger than its binding to the H3K36me3 peptide alone ( K d =36 μM, ref. 3 ). Pulldowns using Y47A mutant of GST-Tudor and the H3K C 36me3-NCP or wild-type GST-Tudor and unmodified NCP showed much weaker associations. In agreement with NMR data, these results indicate that recognition of H3K36me3 is the key requirement for PHF1 Tudor to bind the nucleosome; however, additional contacts with the NCP beyond those with the histone tail contribute to the complex formation. 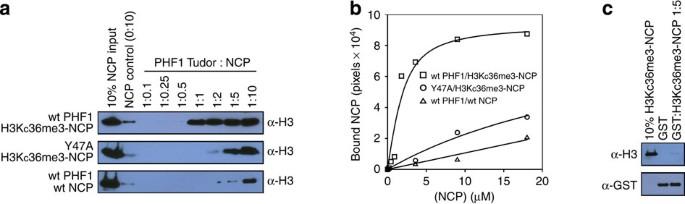Figure 2: Tudor interaction with the nucleosome is dependent on methylation at H3K36. (a) Western analysis of pulldowns of wild-type (wt) GST-Tudor with H3KC36me3-NCP (top) of Y47A GST-Tudor with H3KC36me3-NCP (middle) or wild-type GST-Tudor with the unmodified wild-type NCP (bottom). (b) The representative binding curves shown for each combination of the Tudor domain and NCP. Densitometry analysis of the bound H3KC36me3-NCP reveals an apparent affinity of 1.3±0.5 μM (SD based on three experiments) of wild-type GST-Tudor (squares), and significantly weaker association of the Y47A mutant GST-Tudor with H3KC36me3-NCP (circles) or wild-type Tudor with wild-type nucleosomes (triangles). All experiments were performed in triplicate. (c) Western blot analysis of GST pulldown with H3KC36me3-NCP showing that GST does not bind to H3KC36me3-NCP. Figure 2: Tudor interaction with the nucleosome is dependent on methylation at H3K36. ( a ) Western analysis of pulldowns of wild-type (wt) GST-Tudor with H3K C 36me3-NCP (top) of Y47A GST-Tudor with H3K C 36me3-NCP (middle) or wild-type GST-Tudor with the unmodified wild-type NCP (bottom). ( b ) The representative binding curves shown for each combination of the Tudor domain and NCP. Densitometry analysis of the bound H3K C 36me3-NCP reveals an apparent affinity of 1.3±0.5 μM (SD based on three experiments) of wild-type GST-Tudor (squares), and significantly weaker association of the Y47A mutant GST-Tudor with H3K C 36me3-NCP (circles) or wild-type Tudor with wild-type nucleosomes (triangles). All experiments were performed in triplicate. ( c ) Western blot analysis of GST pulldown with H3K C 36me3-NCP showing that GST does not bind to H3K C 36me3-NCP. Full size image Tudor associates with DS-DNA To explore whether the PHF1 Tudor domain makes contacts other than to the histone tail sequence in the nucleosome, we tested its ability to bind DNA. Titration of a 10 bp DS-DNA fragment into 15 N-labelled Tudor induced substantial chemical shift changes in the protein ( Fig. 3a , first panel). In contrast, titration of a single strand of the same DNA fragment did not lead to resonance perturbations, indicating that this interaction is specific for DS-DNA and likely depends on the presence of a major/minor groove ( Fig. 3a , second panel). Analysis of the chemical shift perturbations (CSPs) afforded a K d of 201 μM for binding of the Tudor domain to the 10 bp DS-DNA. Furthermore, the 601 DNA sequence, which we used to reconstitute the H3K C 36me3-NCP, caused large CSPs in the Tudor domain, which were generally similar in direction to those seen upon addition of the 10 bp DS-DNA; however, the presence of ~14 major/minor grooves in the 601 DNA construct, and thus non-stoichiometric association, precluded a straightforward quantitative analysis of this interaction ( Fig. 3a , third panel). Nevertheless, the pattern of CSPs inferred that the Tudor domain binds to DS-DNA in a non-specific manner. A plot of the resonance perturbations as a function of Tudor residue revealed that the residues involved in the interaction with DNA lay along the β-barrel sides and around the H3K36me3 binding pocket ( Fig. 3b,c ). Subsequent titration of the H3K36me3 peptide into the 10 bp DS-DNA-bound Tudor domain caused additional CSPs in the protein, and the intermediate exchange regime indicated a stronger interaction with H3K36me3 ( Fig. 3d ). Together these data suggest that within the intact NCP the Tudor domain can concomitantly interact specifically with the methylated histone H3 tail as well as non-specifically with the nucleosomal DNA. 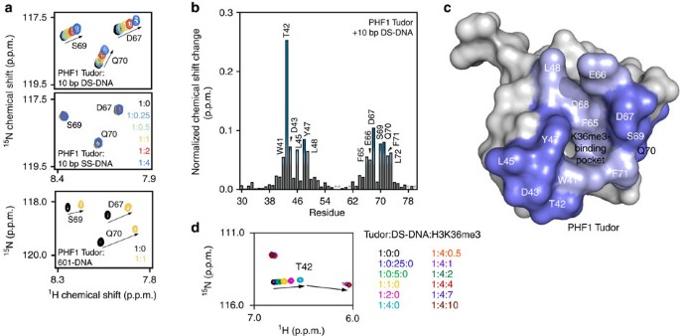Figure 3: Tudor interacts non-specifically with DS-DNA. (a)1H,15N HSQC overlay of Tudor in the presence of increasing concentrations of a 10 bp fragment of DS (top) or single-stranded (middle) DNA or the DS Widom 601 DNA sequence (bottom). (b) A plot of the normalized chemical shift change induced upon titration of the 10 bp DS-DNA fragment as a function of Tudor residue, with changes greater than the average plus1/3and average plus2/3the standard deviation shown in light blue and dark blue, respectively. (c) Residues showing significant chemical shift changes inbare mapped onto a surface representation of Tudor. (d) The Tudor domain binds weaker to DS-DNA and stronger to H3K36me3. Superimposed1H,15N HSQC spectra of the Tudor domain collected upon addition of a 10 bp DS-DNA fragment (fast exchange regime), followed by addition of H3K36me3 peptide (intermediate exchange regime). Molar ratios of Tudor to DNA to peptide are shown to the right. Figure 3: Tudor interacts non-specifically with DS-DNA. ( a ) 1 H, 15 N HSQC overlay of Tudor in the presence of increasing concentrations of a 10 bp fragment of DS (top) or single-stranded (middle) DNA or the DS Widom 601 DNA sequence (bottom). ( b ) A plot of the normalized chemical shift change induced upon titration of the 10 bp DS-DNA fragment as a function of Tudor residue, with changes greater than the average plus 1 / 3 and average plus 2 / 3 the standard deviation shown in light blue and dark blue, respectively. ( c ) Residues showing significant chemical shift changes in b are mapped onto a surface representation of Tudor. ( d ) The Tudor domain binds weaker to DS-DNA and stronger to H3K36me3. Superimposed 1 H, 15 N HSQC spectra of the Tudor domain collected upon addition of a 10 bp DS-DNA fragment (fast exchange regime), followed by addition of H3K36me3 peptide (intermediate exchange regime). Molar ratios of Tudor to DNA to peptide are shown to the right. Full size image The model of the PHF1 Tudor/H3K C 36me3-NCP complex We generated a model of the PHF1 Tudor domain bound to the H3K C 36me3-NCP using the docking program HADDOCK. A three-body docking protocol utilizing Tudor/H3K36me3 (4HCZ), the histone octamer with H3 cut at His39, and DNA (3LZ0) was applied. A total of ~64 K restraints between the octamer and DNA were used, and Pro38 of the H3K36me3 histone peptide was constrained to a bonding distance with His39 of the octamer either near the entry point of DNA or the exit point of DNA. Docking calculations of Tudor at either entry/exit point yielded very similar results, and comparison of the two models suggests that two Tudor domains can simultaneously associate with the NCP symmetrically trimethylated at Lys36 on both H3 tails ( Fig. 4 ). 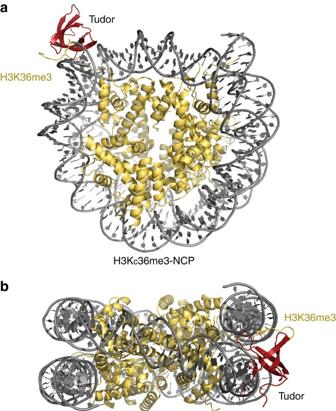Figure 4: A model of the Tudor/H3KC36me3-NCP complex. HADDOCK model of Tudor bound to the H3KC36me3-NCP. The Tudor domain is shown in mauve, nucleosomal DNA in grey and histones in yellow. The Lys36me3 residue is shown as sticks. Docking calculations were performed for Tudor at both histone H3 tails near the entry (a) and exit (b) regions of the DNA. Figure 4: A model of the Tudor/H3K C 36me3-NCP complex. HADDOCK model of Tudor bound to the H3K C 36me3-NCP. The Tudor domain is shown in mauve, nucleosomal DNA in grey and histones in yellow. The Lys36me3 residue is shown as sticks. Docking calculations were performed for Tudor at both histone H3 tails near the entry ( a ) and exit ( b ) regions of the DNA. Full size image The model suggests that Tudor is stabilized at the H3K C 36me3-NCP through concomitant interactions with the trimethylated histone tail and the minor groove and backbone of the nucleosomal DNA ( Fig. 4 ). The Tudor domain is positioned between the two gyres of the DNA superhelix with the hydrophobic patch and β1 and β2 strands aligned with the minor groove of the DNA helical segment nearest the dyad. In addition, there are a few contacts between the residues in and around the Lys36me3 binding pocket and the phosphate backbone of the entry/exit DNA. The model is in good agreement with CSPs observed upon titration of DS-DNA and the H3K C 36me3-NCP, and although the full histone tail was not included in the docking algorithm, the orientation of the residues N-terminal to Lys36me3 suggests that some of the additional CSPs seen upon titration of the H3K C 36me3-NCP may be due to interactions between these histone residues and the Tudor domain in the context of the entire NCP. We also note that during the docking calculation the DNA was extensively restrained on the octamer core. Our numerous attempts to examine the effect of the Tudor association on the NCP breathing dynamics by applying limited or no restraints at the entry/exit ends of DNA have failed. Nevertheless, modelling using the fully restrained NCP shows that the Tudor domain does not lock the DNA into a wrapped position at either orientation, implying that the entry/exit DNA can be readily lifted off the core. Interaction with H3K36me3 stabilizes a more open form of NCP What is the consequence of binding of the PHF1 Tudor domain to H3K36me3 in the NCP? The location of H3K36me3 in the nucleosome readily positions this mark itself, as well as the PHF1 Tudor docking to this PTM, to influence nucleosomal DNA unwrapping/rewrapping or DNA accessibility and binding of regulatory proteins to DNA sites wrapped onto the nucleosome. We therefore investigated the impact of recognition of H3K36me3 by the PHF1 Tudor domain on nucleosome unwrapping and binding of the DNA-specific repressor protein LexA using FRET ( Fig. 5 ). H3K C 36me3-NCPs were prepared with the 147 bp 601 nucleosome positioning sequence, this time with the LexA binding sequence replacing bases 8–27 (601L, Fig. 5a–c ). The Cy3 donor fluorophore was attached to the 5′ end of the 601L DNA molecule adjacent to the LexA site, and the Cy5 acceptor fluorophore was attached to H2A(K119C) ( Fig. 5c ). This positions Cy3 in the proximity of one of the Cy5 fluorophores so that there is significant energy transfer from fully wrapped nucleosomes ( Fig. 5d ), whereas a reduction in FRET efficiency implies a decrease in nucleosome wrapping [21] , [23] . 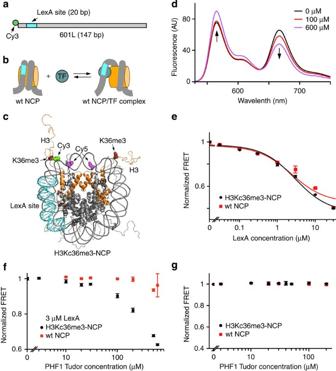Figure 5: PHF1 Tudor binding to the H3KC36me3-NCP stabilizes a more open form of the nucleosome. FRET measurements of the influence of PHF1 Tudor on TF binding. (a) Diagram of the 601L DNA molecule. (b) A two-state model of TF binding to its target site within the nucleosome. (c) Crystal structure of the NCP (PDB ID: 1KX5) that indicates the positions of H3 (orange); MLA at H3K36C (dark red); Cy5 at H2AK119C (purple); Cy3 at the 5′ end of 601L (green); and the LexA target site (cyan). (d) Fluorescence spectra with Cy3–Cy5-labelled H3KC36me3-NCPs with 3 μM of LexA and either 0 μM (black), 10 μM (red) and 600 μM (purple) of PHF1 Tudor. The Cy3 emission increases as the Cy5 emission decreases indicating a decrease in FRET efficiency. (e) FRET efficiencies of LexA titrations with H3KC36me3 (black) and unmodified wild-type nucleosomes (red). FRET efficiencies were done in duplicate and fit to a non-cooperative binding curve with S1/2of 3,000±600 nM and 2,400±900 nM for H3KC36me3 and unmodified wild-type nucleosomes, respectively. (f,g) FRET efficiencies of PHF1 Tudor titrations with (f) and without (g) 3 μM LexA and either H3KC36me3 (black) or unmodified NCPs (red). Error bars represent a standard deviation based on three experiments (PHF1 titrations) or two experiments (LexA titrations). Figure 5: PHF1 Tudor binding to the H3K C 36me3-NCP stabilizes a more open form of the nucleosome. FRET measurements of the influence of PHF1 Tudor on TF binding. ( a ) Diagram of the 601L DNA molecule. ( b ) A two-state model of TF binding to its target site within the nucleosome. ( c ) Crystal structure of the NCP (PDB ID: 1KX5) that indicates the positions of H3 (orange); MLA at H3K36C (dark red); Cy5 at H2AK119C (purple); Cy3 at the 5′ end of 601L (green); and the LexA target site (cyan). ( d ) Fluorescence spectra with Cy3–Cy5-labelled H3K C 36me3-NCPs with 3 μM of LexA and either 0 μM (black), 10 μM (red) and 600 μM (purple) of PHF1 Tudor. The Cy3 emission increases as the Cy5 emission decreases indicating a decrease in FRET efficiency. ( e ) FRET efficiencies of LexA titrations with H3K C 36me3 (black) and unmodified wild-type nucleosomes (red). FRET efficiencies were done in duplicate and fit to a non-cooperative binding curve with S 1/2 of 3,000±600 nM and 2,400±900 nM for H3K C 36me3 and unmodified wild-type nucleosomes, respectively. ( f , g ) FRET efficiencies of PHF1 Tudor titrations with ( f ) and without ( g ) 3 μM LexA and either H3K C 36me3 (black) or unmodified NCPs (red). Error bars represent a standard deviation based on three experiments (PHF1 titrations) or two experiments (LexA titrations). Full size image We first examined the effect of H3K C 36me3 on nucleosome wrapping using LexA and Cy3–Cy5-labelled NCPs. The concentration of LexA required to bind 50% of the nucleosomes (S 1/2 ) is inversely proportional to the probability the LexA target site being unwrapped from the nucleosome for LexA binding [23] ( Fig. 5b ). Thus a reduction of S 1/2 induced by H3K C 36me3 would imply an increase in partial nucleosome unwrapping. Upon titration of LexA into Cy3–Cy5-labelled wild-type NCP or H3K C 36me3-NCP we observed a decrease in FRET, due to LexA binding and stabilization of the unwrapped state. We found the LexA S 1/2 to be 3,000 nM and 2,400 nM for H3K C 36me3 and wild-type nucleosomes, respectively ( Fig. 5e ). The similar S 1/2 values indicate that H3K C 36me3 itself does not directly impact nucleosome unwrapping. We next titrated Tudor into 50 nM of wild-type NCP or H3K C 36me3-NCP in the presence of 3 μM (S 1/2 ) LexA. We found that above 30 μM of PHF1 Tudor, the FRET efficiency is substantially reduced for nucleosomes containing H3K C 36me3, whereas the FRET efficiency for unmodified nucleosomes remains unchanged ( Fig. 5f ). This data indicate that Tudor binding to H3K C 36me3 disturbs the nucleosome, facilitating LexA binding to its target sequence buried within the nucleosome. This ability to facilitate LexA binding was further enhanced when a larger PHF1 construct, containing the Tudor domain and adjacent PHD1 finger, was examined ( Fig. 6a ). Because the PHD1 finger has no effect on binding of the Tudor domain to H3K36me3 ( Fig. 6b ) and shows no histone-binding activity [5] , these results suggest that the increase in size of the NCP-interacting macromolecule produces the greater effect. Addition of PHF1 Tudor to the H3K C 36me3-nucleosomes in the absence of LexA resulted in no significant change in the FRET efficiency, implying that the presence of the DNA-binding target protein is essential for the enhancement of the DNA accessibility ( Fig. 5g ). Together, our findings support the previously proposed idea that transcription factor (TF) binding to a target site may expedite TF binding to a second target site further into the nucleosome [24] , [25] , and provide the first example of such a heteromolecular augmentation ( Fig. 6c ). 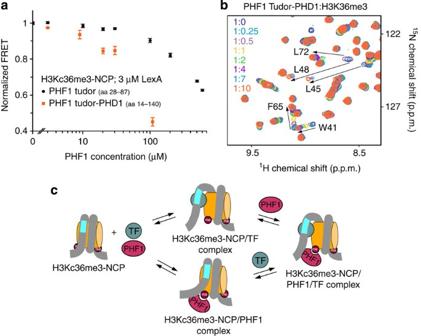Figure 6: The larger PHF1 construct containing Tudor and PHD1 further enhances LexA binding. (a) FRET efficiencies of the PHF1 Tudor (black) and Tudor-PHD1 (orange) titrations with H3KC36me3 nucleosomes in the presence of 3 μM LexA. Error bars represent a standard deviation based on three experiments. (b) Superimposed1H,15N HSQC spectra of PHF1 Tudor-PHD1 recorded as H3K36me3 peptide was titrated in. An almost identical pattern of chemical shift changes was observed in the Tudor domain linked to the PHD1 finger, as compared with the changes seen in this domain alone (see ref.3). Arrows indicate most notable changes. Resonances corresponding to the PHD1 finger were unperturbed, implying that PHD1 is not involved in this interaction. (c) Four-state model of PHF1 Tudor and LexA binding to nucleosomes. Figure 6: The larger PHF1 construct containing Tudor and PHD1 further enhances LexA binding. ( a ) FRET efficiencies of the PHF1 Tudor (black) and Tudor-PHD1 (orange) titrations with H3K C 36me3 nucleosomes in the presence of 3 μM LexA. Error bars represent a standard deviation based on three experiments. ( b ) Superimposed 1 H, 15 N HSQC spectra of PHF1 Tudor-PHD1 recorded as H3K36me3 peptide was titrated in. An almost identical pattern of chemical shift changes was observed in the Tudor domain linked to the PHD1 finger, as compared with the changes seen in this domain alone (see ref. 3 ). Arrows indicate most notable changes. Resonances corresponding to the PHD1 finger were unperturbed, implying that PHD1 is not involved in this interaction. ( c ) Four-state model of PHF1 Tudor and LexA binding to nucleosomes. Full size image In the past few years, our knowledge of how reader domains bind PTMs on histone tails has grown significantly; however, very few studies have investigated the mechanism of these associations in the context of the full nucleosome [6] , [7] , [8] , [9] , [10] , [26] . We have previously determined the structural basis for the interaction of the PHF1 Tudor domain with a H3K36me3 peptide [3] . In this work, we characterize binding of PHF1 Tudor to the intact H3K C 36me3-NCP. We find that in addition to its histone-binding capabilities, PHF1 Tudor interacts non-specifically with a DS-DNA. The multiple interactions may account for the higher affinity of Tudor for the H3K C 36me3-NCP as compared with its affinity for the histone H3K36me3 peptide. Dual association with H3K36me3 and nucleosomal DNA has recently been reported for the PWWP domain of LEDGF/PSIP1 (refs 8 , 9 ). Whereas PWWP binds to a DNA fragment or the H3K36me3 peptide with low affinities ( K d of ~150 μM and 11–17 mM, respectively), bipartite binding to the H3K C 36me3-nucleosome results in a strong interaction ( K d of ~1.5 μM) [8] , [9] . Particularly, interaction with nucleosomal DNA was found to be responsible for a ~10 4 -fold enhancement in binding affinity and drives the recognition of the H3K C 36me3-NCP [8] , [9] . Much like PWWP, the PHF1 Tudor domain binds to the H3K C 36me3-NCP with a ~1.3 μM affinity; however, its tight association with the H3K36me3 peptide alone ( K d of ~36 μM) suggests that the recognition of methylated Lys36 is the driving force for the Tudor–H3K C 36me3-NCP interaction. Nucleosomes have been shown to undergo spontaneous conformational fluctuations, in which a stretch of the entry/exit point DNA lifts off the histone core, providing transient access to the occluded regions of DNA for DNA-binding regulatory proteins and protein complexes [20] , [21] , [22] , [27] . The unwrapping and following rewrapping processes are fast, with spontaneous opening occurring within ~250 ms, and are widespread, with the DNA ends being unwrapped in 1–5% of NCPs at any point [20] , [21] , [22] . On average, the NCP stays unwrapped only ~10–50 ms before rewrapping [20] . Within this short interval, some regulatory proteins are able to bind their respective target DNA sequences, but this time is not sufficient for RNA polymerase II (Pol II) to advance by even 1 bp [20] . It takes on average ~6–7 s for Pol II to elongate through the nucleosome, or ~2 s to process a ~40–50 bp linker DNA [20] . Consequently, the NCP undergoes many cycles of rapid unwrapping and rewrapping before Pol II fully moves onto the nucleosome. Our data demonstrate that interaction of the PHF1 Tudor domain with the H3K C 36me3-NCP facilitates binding of LexA to its target DNA sequence buried within the nucleosome, which is inaccessible in the fully wrapped NCP. This indicates a shift in equilibrium towards a more open form of the nucleosome and hindering the rewrapping event in the presence of the DNA-binding protein. HADDOCK analysis of the Tudor–H3K C 36me3-NCP interaction suggests a mechanism for this shift. Because the Tudor domain binds H3K36me3 between the two gyres of the DNA superhelix and does not lock the DNA entry point, once the DNA lifts off, the bound PHF1 Tudor may sterically preclude rapid DNA rewrapping, thus increasing the DNA accessibility to its ligand protein. As the H3K36me3 mark is found in actively transcribed gene bodies, it will be interesting to explore the effect of the PHF1–H3K36me3 interaction on the elongation activity of Pol II and whether this effect can be altered by chromatin fibre density and nucleosome positioning. Furthermore, it will be important to establish the significance of recognition of one H3K36me3 mark or two H3K36me3 marks on a single NCP. Last, future studies are also necessary to determine whether the nucleosomal changes imparted by Tudor association with H3K36me3 may have a role in PHF1 functions, particularly in modulating the methyltransferase activity of PRC2 and mediating PHF1 accumulation at DNA damage sites. DNA constructs and protein purification The wild-type PHF1 Tudor domain (residues 14–87 or residues 28–87) and Tudor-PHD1 (restudies 14–140) were cloned from full-length hPHF1 (obtained from Open Biosystems). Point mutant Y47A was generated by site-directed mutagenesis using the Stratagene QuickChange XL kit. Wild-type and mutant proteins were expressed in Escherichia coli BL21(DE3) pLysS cells grown in LB or 15 NH 4 Cl-supplemented M9-minimal media (grown in D 2 O for purposes of NMR nucleosome binding studies) and induced with IPTG (isopropyl-β- D -1-thiogalactopyranoside). Bacteria were harvested by centrifugation and lysed by sonication. The unlabelled, 15 N-labelled and 2 D/ 15 N-labelled GST-fusion proteins were purified using glutathione Agarose 4B beads (Fisher). The GST tag was either cleaved with Prescission protease, or left for the purposes of pulldowns, in which case the GST-fusion protein was eluted off the glutathione Agarose beads using 0.05 M reduced L -glutathione (Sigma Aldrich). Xenopus histone proteins H2A, H2B, H3C110A, H3K36C/C110A and H4 were expressed in E. coli BL21(DE3) pLysS cells grown in 2XYT media and induced with IPTG. Bacteria were harvested by centrifugation and lysed by sonication. Proteins were extracted from inclusion bodies, purified over ion exchange resin and lyophilized. Thirty-two repeats of the 601 Widom sequence were cloned into the pJ201 plasmid. The plasmid was purified in high yield primarily following the protocol outlined in ref. 28 . The individual sequences were released from the plasmid using EcoRV and purified away from the parental plasmid using polyethylene glycol precipitation [29] . MLA generation Histone H3(C110A)K36C point mutant was generated by site-directed mutagenesis using the Stratagene QuickChange XL kit and purified as described above. The histone H3K C 36me3 was generated by alkylation of H3K36C with (2-bromoethyl) trimethylammonium bromide following the protocol outlined in ref. 30 . After desalting, the protein was dialysed into water and re-lyophilized. HADDOCK modelling HADDOCK modelling was performed via the webserver interface [31] , [32] . The crystal structure Tudor in complex with the H3K36me3 peptide (PDBID: 4HCZ) including peptide residues 31–38 was docked onto the 601-NCP crystal structure (PDBID: 3LZ0) with the H3 tail cut at His39. A three-body docking protocol was followed, in which the histone octamer was taken as a single chain, the nucleosomal DNA as the second chain and the Tudor in complex with H3K36me3 peptide as the third chain. Extensive unambiguous restraints were generated between the histone octamer and DNA and the peptide residue Pro38 and the histone octamer residue His39 were restrained to a bonding distance. Semi-flexibility options for the DNA and octamer were set to ‘none’, and the Tudor/peptide was set to automatic. The final model was chosen which had the best HADDOCK score and best fit for all restraints. In the final structure, a covalent bonding distance was enforced between Pro38 and His39. Calculations were run for Tudor at both of the histone H3 tails in the NCP. Nucleosome reconstitution Equimolar ratios of H2A, H2B, H4 and either H3(C110A) or H3(C110A)K C 36me3 were mixed and refolded into 2 M NaCl, 10 mM Tris pH 7.5 and 5 mM β-mercaptoethanol to form the histone octamer [28] . The octamer was purified by size exclusion chromatography on a sephacryl S-300 column. Purified octamer was mixed at a 1.2:1 ratio with purified 601 DNA and desalted according to protocol [28] into a final buffer of 20 mM Tris pH 7.5, 150 mM NaCl and 5 mM β-mercaptoethanol. The nucleosome was further purified from free DNA by sucrose gradient. Pulldown assays GST-fusion PHF1 Tudor was incubated with reconstituted H3K C 36me3- or wild-type nucleosomes in binding buffer containing 20 mM Tris (pH 7.5), 150 mM NaCl and 0.2% Triton for 2 h at 4 °C (ref. 8 ). Glutathione-agarose beads were added and further incubated for 1 h at 4 °C. Free nucleosome was washed away by washing 4X with 20 mM Tris (pH 7.5), 275 mM NaCl and 0.2% Triton. Bound nucleosome was detected by western blot using an anti-H3 antibody (1:3,000 dilution) (Abcam, AB1791). A control of nucleosome with beads alone (at the equivalent of a 0:10 molar ratio) was used to assess for non-specific binding. Blots were analysed using ImageJ and normalized to account for non-specific binding. The apparent K d was calculated using the equation: where [ L ] is concentration of the nucleosome, [ P ] is the concentration of Tudor, Pixels is the normalized pixel count calculated in ImageJ and Pixels max is the count at saturation. For control, GST pulldown with H3K C 36me3-NCP was analysed using western blot, which was first probed with an anti-H3 antibody (Abcam ab1791) and then stripped with strip buffer (1.5% (w/v) glycine, 0.1% (w/v) SDS, 1% Tween-20, pH 2.2) for an hour, re-blocked and probed with anti-GST-horseradish peroxidase antibody (GE Life Sciences RPN1236V) overnight. NMR spectroscopy NMR experiments were collected on Varian 900 MHz and 600 MHz spectrometers equipped with a cryogenic probes at the University of Colorado School of Medicine NMR core facility. 1 H, 15 N HSQC or TROSY-HSQC experiments were carried out at 298 K (peptide and 10 bp DNA) or 310 K (nucleosome and 601 DNA) on 15 N- or 2 D/ 15 N-labelled Tudor (wild type or mutant) or Tudor-PHD1 in 20 mM Tris pH 6.8 and 150 mM NaCl. Spectra were recorded in the presence of increasing concentrations of H3K36me3 peptide (synthesized by the University of Colorado Peptide Core Facility), 10 bp SS-DNA, 10 bp DS-DNA, 601 DNA or reconstituted nucleosomes. K d value for the Tudor–DS-DNA interaction was calculated by a nonlinear least-squares analysis in Kaleidagraph using the equation: where [ L ] is the concentration of DS-DNA, [ P ] is the concentration of the protein, Δ δ is the observed normalized chemical shift change and Δ δ max is the normalized chemical shift change at saturation, calculated as where δ is the chemical shift in p.p.m. Nucleosome and LexA preparation for FRET measurements Nucleosomal DNA, 601L was prepared by PCR from a plasmid containing the LexA binding site at bases 8–27 with the Cy3-labelled oligonucleotide, Cy3-CTGGAGATACTGTATGAGCATACAGTACAATTGGTC and the unlabelled oligonucleotide, ACAGGATGTATATATCTGACACGTGCCTGGAGACTA. The Cy3-labelled oligonucleotide was labelled using a Cy3-NHS esther (GE Healthcare) at a 5′ amino group and purified by reverse phase HPLC on a 218TPTM C18 (Grace/Vydac) column. Xenopus histones were expressed and purified as in ref. 28 . All H3 histones contained the H3C110A mutation. LexA was expressed and purified by known methods. H3K C 36me3 was prepared as reported [30] , [33] . Briefly, recombinant H2AK119C and H2B were refolded into heterodimer and then labelled with Cy5-maleamide (GE Healthcare). Heterodimer was first reduced in 10 mM tris(2-carboxyethyl)phosphine (TCEP) pH 7.1 for 0.5 h, and then dialysed against 5 mM sodium PIPES pH 6.1, 2 M NaCl. After reclaiming, heterodimer was purged under argon at 4 °C for 30 min, and 2 M HEPES pH 7.1 was bubbled with argon at 4 °C for 5 min. The Cy5-maleamide was dissolved in anhydrous dimethylformamide to a concentration of 22 mM and added to heterodimer in a 25-fold molar excess. Sample was gently rotated for 1 h at room temperature and overnight at 4 °C. The heterodimer was then purified by gel filtration on a Superdex 200 column. The labelling efficiency for the reaction was 88% as measured by ultraviolet–visible absorption. H3K C 36me3 and unmodified H3 were separately refolded with H4 into tetramer. H3–H4 tetramer in 0.5 mM potassium phosphate (pH 7.5) with 2 M NaCl was then combined with 10% excess Cy5-labelled H2AK119C-H2B heterodimer in 5 mM pipes (pH 6.1) with 2 M NaCl and incubated at 4 °C overnight to form histone octamer. The resulting octamer was purified by gel filtration on a Superdex 200 column. Nucleosomes were reconstituted by double dialysis with 10% excess 601L DNA into 0.5 mM potassium phosphate (pH 7.5) with 1 mM benzamidine (BZA). Reconstituted nucleosomes were purified by 5–30% sucrose gradient. FRET measurements All FRET efficiency measurements were determined from spectra acquired by a Horiba Scientific Fluoromax 4. Samples were excited at 510 and 610 nm and the photoluminescence spectra were measured from 530 to 750 nm and 630 to 750 nm for donor and acceptor excitations, respectively. Each wavelength was integrated for 1 s, and the excitation and emission slit width were set to 5 nm with 2 nm emission wavelength steps. FRET measurements were computed through the (ratio) A method. LexA titrations were carried out in 75 mM NaCl, 0.1 mM potassium phosphate pH 7.5, 11.5 mM Tris–HCL pH 7.5, 0.00625% IGEPAL and 0.00625% TWEEN20 with 10 nM nucleosomes. PHF1 Tudor and Tudor-PHD1 titrations were carried out with or without 3 μM LexA in 75 mM NaCl, 62.5 μM potassium phosphate pH 7.5, 15.25 mM Tris pH 7.5, 0.00625% IGEPAL, 0.00625% TWEEN20 with 50 nM nucleosomes. The nucleosome concentration was increased to 50 nM to compensate for increased background caused by the addition of PHF1. The change in nucleosome concentration does not impact the FRET measurements because the (ratio) A method is insensitive to fluorescence intensity, and does not impact LexA and PHF1 Tudor binding as both concentrations are significantly below the micromolar concentrations required for LexA and PHF1 Tudor binding. FRET values in each titration were normalized to the FRET efficiency in the absence of the titrant. Titrations were fit to E =( E f − E 0 )/(1+( S ½ / C )+ E 0 , where E is the FRET efficiency at concentration C of the titrant, E 0 the efficiency in the absence of the titrant, E f the efficiency at high titrant concentration and S ½ is the inflection point. Errors in Figs 5 and 6 represent a standard deviation based on three experiments (PHF1 titrations) or two experiments (LexA titrations). Errors for fits represent 68% confidence bounds. How to cite this article: Musselman, C. A. et al. Binding of PHF1 Tudor to H3K36me3 enhances nucleosome accessibility. Nat. Commun. 4:2969 doi: 10.1038/ncomms3969 (2013).